MazF ribonucleases promoteMycobacterium tuberculosisdrug tolerance and virulence in guinea pigs Toxin–antitoxin (TA) systems are highly conserved in members of the Mycobacterium tuberculosis (Mtb) complex and have been proposed to play an important role in physiology and virulence. Nine of these TA systems belong to the mazEF family, encoding the intracellular MazF toxin and its antitoxin, MazE. By overexpressing each of the nine putative MazF homologues in Mycobacterium bovis BCG, here we show that Rv1102c (MazF3), Rv1991c (MazF6) and Rv2801c (MazF9) induce bacteriostasis. The construction of various single-, double- and triple-mutant Mtb strains reveals that these MazF ribonucleases contribute synergistically to the ability of Mtb to adapt to conditions such as oxidative stress, nutrient depletion and drug exposure. Moreover, guinea pigs infected with the triple-mutant strain exhibits significantly reduced bacterial loads and pathological damage in infected tissues in comparison with parental strain-infected guinea pigs. The present study highlights the importance of MazF ribonucleases in Mtb stress adaptation, drug tolerance and virulence. Toxin–antitoxin (TA) systems are mostly bicistronic genetic elements comprising antitoxin and toxin genes. These were initially discovered as plasmid maintenance systems and have been subsequently identified in various bacterial and archaeal genomes [1] , [2] , [3] . Many families of TA systems have been identified and based on the mode of action and chemical nature of the antitoxin; these have been broadly classified into five different classes [4] . The RNA antitoxin components of Type I and Type III TA systems inactivate their cognate toxin partner by either antisense regulation or protein–RNA interactions. Type II, IV and V TA systems feature a protein antitoxin that inactivates the toxin by (i) interacting with the toxin partner, (ii) binding to the toxin target sequence or (iii) cleaving the toxin messenger RNA. However, under conditions of stress such as starvation, guanosine pentaphosphate- and inorganic phosphate-mediated degradation of an antitoxin leads to activation of cognate toxin, resulting in inhibition of cellular metabolism [5] . This toxin-mediated growth arrest allows the bacteria to withstand unfavourable environmental conditions [6] . TA systems are widespread in bacterial genomes and contribute to prokaryotic stress adaptation and the formation of persister cells and biofilms [1] , [7] , [8] , [9] . The toxin components of the TA modules exert their effects in different ways by targeting essential cellular functions such as DNA replication, protein synthesis, cell division, peptidoglycan biosynthesis and ribosome assembly; however, RNA cleavage is the most prevalent mode of action [10] , [11] , [12] , [13] , [14] , [15] , [16] . These ribonucleases cleave RNA in either a ribosome-dependent (for example, RelE, HigB and YoeB) or ribosome-independent manner (for example, MazF, ToxN and VapC) [17] , [18] . In Escherichia coli , one of the most well-characterized TA modules is mazEF , an operon that encodes the intracellular toxin MazF and its cognate antitoxin MazE. MazF toxins cleave mRNA at 3-, 5- or 7-base recognition sequences in different bacteria and have been implicated in controlling cellular responses to various adverse conditions encountered by the bacteria in the host. The E. coli MazF protein cleaves both mRNA and 16S ribosomal RNA, and is proposed to generate a subpopulation of stress ribosomes, thereby enabling the translation of leaderless transcripts [19] . MazEF systems in E. coli are activated on exposure to numerous stress conditions in an extracellular death factor-dependent manner [20] , [21] , [22] . In E. coli , MazF-mediated drug-induced persistence is RecA independent, but dependent on ClpP and Lon proteases [23] . TA systems are ubiquitous in mycobacteria and are highly conserved among members of the Mycobacterium tuberculosis (Mtb) complex, which includes Mtb , Mycobacterium bovis , Mycobacterium africanum , Mycobacterium cannetti and Mycobacterium microti . The Mtb genome contains an unusual abundance of TA systems (>80 putative pairs), most of which belong to the mazEF , relBE , parDE , ccdAB , higBA or vapBC families [24] . These systems are differentially regulated under various stress conditions and the presence of free toxin induces a quasi-dormant state, a metabolic condition identical to that of dormant bacilli. MazF and RelE homologues from Mtb have been extensively characterized biochemically and possess ribonuclease activity. MazF homologues from Mtb exhibit varying substrate specificities; Rv1991c (MazF6), Rv2801c (MazF9) and Rv1495 (MazF4) cleave single-stranded RNA at U ↓ CCUU, U ↓ AC and U ↓ CGCU, respectively [25] , [26] , [27] . In addition to mRNA, Rv1102c (MazF3) also cleaves 23S rRNA at the UU ↓ CCU site and contributes to the formation of both kanamycin- and gentamycin-tolerant persisters of Mycobacterium smegmatis ( Msm ) [28] , [29] . RNA sequencing studies revealed that MazF6 cleaves 23S rRNA within the helix/loop 70 and 16S rRNA at the anti-Shine Dalgarno sequence [27] . Besides ribonuclease activity, MazF4 also affects bacterial survival by modulating DNA topoisomerase activity [30] . The overexpression of Rv2866 (RelE2) results in cell elongation in Msm and RelE toxins also contribute to drug tolerance in vitro [31] , [32] . The HigB toxin targets tmRNA, IdeR and Zur-regulated transcripts, and its activity is regulated by a SecB-like chaperone, Rv1957 (refs 33 , 34 ). VapC toxins regulate Mtb growth via mRNA or 23S rRNA cleavage, or by regulating glycerol consumption rates in vitro [35] , [36] , [37] . Some of these VapC homologues are redundant in nature and Msm with no functional TA system exhibits a severe growth defect in complex media [35] , [38] . Despite this extensive biochemical characterization, the functional significance of MazF homologues in the stress adaptation, drug tolerance and virulence of Mtb is unknown. In the present study, we report that overexpression of MazF3, MazF6 and MazF9 inhibits bacterial growth and these mazEF TA systems are differentially regulated under various stress conditions. The construction of various MazF-deficient strains reveals that the simultaneous deletion of these ribonucleases impairs the survival of Mtb under oxidative stress, under nutrient-limiting conditions and in macrophages. We also demonstrate that MazF ribonucleases contribute to in vitro persistence and in vivo virulence. Expression of MazF3, MazF6 and MazF9 inhibit Mtb growth The Mtb genome encodes nine MazF homologues. These toxins appear to be co-transcribed with their cognate antitoxins. The MazF toxins and MazE antitoxins share 20–30% identity among themselves. To understand the biological role of mazEF TA systems in Mtb , we first sought to determine the effect of MazF overexpression on mycobacterial growth using anhydrotetracycline (Atc)-inducible vectors. The overexpression of three homologues, MazF3, MazF6 and MazF9, led to growth inhibition of both M. bovis BCG and Mtb compared with a vector-harbouring strain ( Fig. 1a,b ). Overexpression of MazF3, MazF6 and MazF9 reduced bacterial loads by ~8.0-, 22.0- and 18.0-fold, respectively, compared with the vector-harbouring strain at day 7 post induction (paired (two-tailed) t -test, P <0.05; Fig. 1b ). This observed growth defect was bacteriostatic, as no decrease in bacterial counts was observed and these bacteria were able to regrow on removal of inducer ( Fig. 1b ). The overexpression of the remaining MazF homologues, Rv0456a (MazF1), Rv0659c (MazF2), MazF4, Rv1942c (MazF5), Rv2063a (MazF7) and Rv2274 (MazF8) did not inhibit M. bovis BCG growth ( Fig. 1a ). The percentage of SYTO-9-stained live bacilli and the ability to generate a proton-motive force were comparable in M. bovis BCG strains harbouring pTE-mcs1 , pTE-mazF3 , pTE-mazF6 or pTE-mazF9 at both day 2 and day 3 post induction ( Supplementary Fig. 1a,b ). As the overexpression of MazF3, MazF6 and MazF9 inhibited bacterial growth, further experiments were performed to elucidate their role in Mtb physiology. 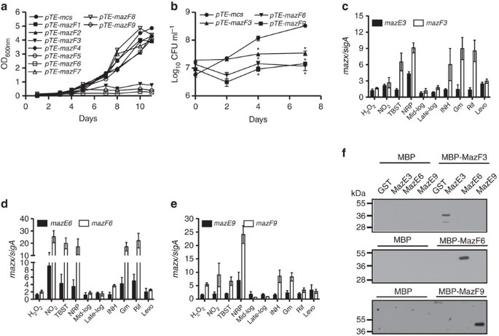Figure 1: Effect of overexpression of MazF toxins on mycobacterial growth. M. bovisBCG (a) orMtbH37Rv (b) were transformed with Atc-induciblepTE-mcs1or its derivatives by electroporation. The effect of MazF toxin overexpression on mycobacterial growth was assayed by measuring either OD600nm(a) or viable bacterial counts (b). The data presented inaandb(mean±s.e.) are representative of three independent experiments. Significant differences were observed for the indicated groups (paired (two-tailed)t-test, *P<0.05). (c–e) Measurement of toxin and antitoxin transcript levels by quantitative RT–PCR (qRT–PCR). For qRT–PCR analysis, mRNA was isolated from early-log, mid-log, late-log and NRP cultures ofMtb. For stress experiments, early-log phase cultures were exposed to oxidative (5 mM H2O2), nitrosative (5 mM NO2) or various drugs for 6 h or nutritional (TBST) for 4 days. qRT–PCR was performed and the relative expression of toxins and antitoxins was calculated after normalization tosigAlevels. The data presented are the mean±s.e. of the transcripts obtained from at least three independent experiments. (f) Interaction between cognate TA proteins. Purified proteins (MBP only, MBP-tagged toxins, GST only, GST-tagged antitoxins) were incubated with pre-equilibrated amylose resin for 2 h, followed by washing with ice-cold binding buffer. The protein complexes bound to amylose resin were resolved by 12.5% SDS–PAGE and analysed by immunoblot analysis using anti-GST antibody. The data shown are representative of two independent experiments. The full blots are shown inSupplementary Fig. 2. Figure 1: Effect of overexpression of MazF toxins on mycobacterial growth. M. bovis BCG ( a ) or Mtb H37Rv ( b ) were transformed with Atc-inducible pTE-mcs1 or its derivatives by electroporation. The effect of MazF toxin overexpression on mycobacterial growth was assayed by measuring either OD 600nm ( a ) or viable bacterial counts ( b ). The data presented in a and b (mean±s.e.) are representative of three independent experiments. Significant differences were observed for the indicated groups (paired (two-tailed) t -test, * P <0.05). ( c – e ) Measurement of toxin and antitoxin transcript levels by quantitative RT–PCR (qRT–PCR). For qRT–PCR analysis, mRNA was isolated from early-log, mid-log, late-log and NRP cultures of Mtb . For stress experiments, early-log phase cultures were exposed to oxidative (5 mM H 2 O 2 ), nitrosative (5 mM NO 2 ) or various drugs for 6 h or nutritional (TBST) for 4 days. qRT–PCR was performed and the relative expression of toxins and antitoxins was calculated after normalization to sigA levels. The data presented are the mean±s.e. of the transcripts obtained from at least three independent experiments. ( f ) Interaction between cognate TA proteins. Purified proteins (MBP only, MBP-tagged toxins, GST only, GST-tagged antitoxins) were incubated with pre-equilibrated amylose resin for 2 h, followed by washing with ice-cold binding buffer. The protein complexes bound to amylose resin were resolved by 12.5% SDS–PAGE and analysed by immunoblot analysis using anti-GST antibody. The data shown are representative of two independent experiments. The full blots are shown in Supplementary Fig. 2 . Full size image Differential regulation of Mtb mazEF TA modules TA systems have been implicated in enabling Mtb to adapt and respond to various adverse conditions encountered in the host. Next, we quantified the relative levels of mazE3 , mazF3 , mazE6 , mazF6 , mazE9 and mazF9 transcripts under various growth conditions and on exposure to various stresses or drugs. The transcript levels of these genes were normalized to the transcript level of sigA , a housekeeping gene, and were compared with their baseline transcription levels in untreated bacteria. Under oxidative stress, mazF9 mRNA levels were upregulated by 5.5-fold, whereas no differences were observed in the transcript levels of mazF3 and mazF6 ( Fig. 1c–e ). The transcription of mazF6 and mazF9 was induced by 25.0- and 9.0-fold, respectively, in Mtb exposed to nitrosative stress ( Fig. 1d,e ). Mtb must adapt to nutrient-limiting and hypoxic conditions to remain dormant and persist in the host. Compared with untreated bacteria, the transcript levels of mazF3 , mazF6 and mazF9 were upregulated by 6.5-, 20.0- and 6.7-fold, respectively, in 1 × tris buffered saline tween 80 (TBST)-treated cultures, and these levels were increased by ~9.1-, 17.1- and 24.1-fold, respectively, in the non-replicative persistence (NRP) state ( Fig. 1c–e ). TA systems are upregulated in persisters and have been described as terminal effectors of bacterial persistence [39] , [40] . Therefore, we next quantified the transcript levels of mazE3 , mazF3 , mazE6 , mazF6 , mazE9 and mazF9 in Mtb treated with inhibitors of DNA replication (levofloxacin, (Levo)), cell wall biosynthesis (isoniazid (INH)), transcription (rifampicin (Rif)) or translation (gentamycin (Gm)). Similar to results obtained with stress-exposed cultures, exposure to drugs with different mechanism of action caused differential effects on transcription of these genes: mazF3 mRNA levels were induced by 6.0-, 8.9- and 8.5-fold by INH, Gm and Rif, respectively; mazF6 mRNA levels were upregulated by 3.6-, 17.1- and 22.1-fold by INH, Gm and Rif, respectively; and transcription of mazF9 was induced by 8.5- and 8.2-fold by INH and Gm, respectively ( Fig. 1c–e ). None of these mazF homologues were upregulated in response to exposure to Levo ( Fig. 1c–e ). Consistent with observations of other TA systems, we also observed relative abundance of maz F transcripts in comparison with mazE transcripts ( Fig. 1c–e ) [32] , [41] , [42] . Compared with early log phase bacteria, no differences were observed in the transcript levels of mazE3 , mazF3 , mazE6 , mazF6 , mazE9 and mazF9 in mid-log and late-log growth stages ( Fig. 1c–e ). These results suggest that mazEF TA systems are differentially regulated on the exposure of Mtb to various stress conditions and drugs. MazF toxins show specificity for their cognate antitoxins We next investigated the specificity of the interactions between the MazF toxins and their cognate antitoxins. To examine protein–protein interactions, maltose binding protein (MBP)-tagged toxins and glutathione S -transferase (GST)-tagged antitoxins were purified to >95% purity and subjected to in vitro pull-down assays. Immunoblot analysis with α-GST revealed specific interactions between cognate MazF toxins and MazE antitoxins ( Fig. 1f and Supplementary Fig. 2 ). In contrast to previous reports [43] , we did not observe any interaction between non-cognate MazF toxins and MazE antitoxins ( Fig. 1f ). Generation of various MazF-deficient Mtb mutant strains A major challenge in understanding the role of TA systems in bacterial physiology and virulence is the redundancy of these systems. The construction of an Rv1102c ( ΔmazF3 ) knockout strain and its characterization in a murine model of tuberculosis has been reported [32] . In the present study, various single-, double- and triple-mutant strains of Mtb were constructed using temperature-sensitive mycobacteriophages ( Supplementary Fig. 3 ). The replacement of MazF3, MazF6 or MazF9 by various antibiotic-resistance genes in their respective mutant strains was confirmed by PCR using gene-specific primers ( Fig. 2a–c and Supplementary Note 1 ). The event of homologous recombination was confirmed by sequencing of PCR amplicons obtained from the mutant strains. We also confirmed the deletion of these ribonucleases in the genomes of the mutant strains by real-time PCR (reverse transcriptase PCR (RT–PCR)) analysis ( Fig. 2d–f ). Next, we quantified the transcript levels of the antitoxins in these mutant strains by RT–PCR, which revealed that the transcript levels of mazE3 were similar in the parental and mutant strains ( Fig. 2d ). However, mazE6 and mazE9 transcript levels were significantly increased by 13.0- and 40.0-fold, respectively, in the triple-mutant strain compared with the parental strain ( Fig. 2e,f , paired (two-tailed) t -test, P <0.05). RT–PCR analysis revealed that the mazE6 transcript levels were similar in the parental, ΔmazF3 , ΔmazF9 and ΔmazF3Δ9 strains. However, mazE9 transcript levels were increased by ~40.0-fold in both the ΔmazF9 and ΔmazF3Δ9 strains compared with the parental strain ( Fig. 2e,f , paired (two-tailed) t -test, P <0.05). As mazE6 and mazE9 transcript levels were increased in the triple-mutant strain, we investigated whether MazF6 and MazF9 cleave mazE6 and mazE9 mRNA, respectively. As shown in Supplementary Fig. 4 , we observed that MazF6 and MazF9 cleave the transcripts of their cognate antitoxins in vitro. As expected, no degradation of mazE6 and mazE9 mRNA was observed in the presence of GST protein and GST-tagged antitoxins ( Supplementary Fig. 4a,b ). These results suggest of a feedback mechanism where mazEF6 and mazEF9 TA systems are regulated at the posttranscriptional level. 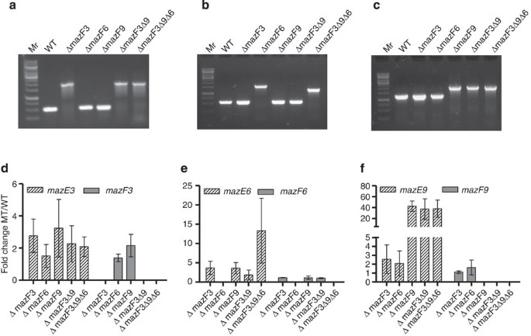Figure 2: Characterization of various mutant strains by PCR and quantitative RT–PCR analysis. Various single-, double- and triple-mutant strains were constructed using temperature-sensitive mycobacteriophages. The disruption ofmazF3(a),mazF6(b) andmazF9(c) in the respective single-, double- and triple-mutant strains was confirmed by PCR using locus-specific primers. (d–f) For RT–PCR analysis, mRNA was extracted from various strains grown until mid-log phase, and cDNA was prepared from DNase I-treated mRNA using Superscript III reverse transcriptase. The synthesized cDNA was subjected to PCR using gene-specific primers. The relative expressions of the toxins and antitoxins were calculated after normalization to the levels ofsigA. The data depicted are the fold change in the mutant strains relative to the wild-type strain and are the mean±s.e. of three independent experiments. Figure 2: Characterization of various mutant strains by PCR and quantitative RT–PCR analysis. Various single-, double- and triple-mutant strains were constructed using temperature-sensitive mycobacteriophages. The disruption of mazF3 ( a ), mazF6 ( b ) and mazF9 ( c ) in the respective single-, double- and triple-mutant strains was confirmed by PCR using locus-specific primers. ( d – f ) For RT–PCR analysis, mRNA was extracted from various strains grown until mid-log phase, and cDNA was prepared from DNase I-treated mRNA using Superscript III reverse transcriptase. The synthesized cDNA was subjected to PCR using gene-specific primers. The relative expressions of the toxins and antitoxins were calculated after normalization to the levels of sigA . The data depicted are the fold change in the mutant strains relative to the wild-type strain and are the mean±s.e. of three independent experiments. Full size image MazF mediate stress adaptation and intracellular survival To investigate the role of MazF3, MazF6 and MazF9 in Mtb growth in vitro , we compared the growth characteristics of the parental and mutant strains. The wild-type and mutant strains exhibited similar growth patterns in liquid media and similar colony morphology on Middlebrook (MB) 7H11 plates ( Supplementary Fig. 5a–c ). Mtb can establish a chronic infection in the host by adapting to the various stress conditions it encounters in the host. As the mazEF TA systems were differentially regulated under the conditions tested in vitro , we evaluated the survival of the parental and mutant strains on exposure to oxidative, nitrosative, nutrient-limiting or low-oxygen stress conditions. The deletion of MazF3, MazF6 and MazF9 ribonucleases in the Mtb genome did not affect survival under nitrosative stress conditions ( Fig. 3a ). However, compared with the parental strain, the triple-mutant strain was ~18.0-fold more susceptible to killing under oxidative stress conditions ( Fig. 3b , paired (two-tailed) t -test, P <0.05). This susceptibility was only specific to the triple-mutant strain; the parental, single-mutant and double-mutant strains survived at comparable levels under these conditions ( Fig. 3b ). In agreement with the induction of mazEF TA systems under nutrient-limiting conditions, ΔmazF3 , ΔmazF9 , ΔmazF3Δ9 and ΔmazF3Δ9Δ6 exhibited survival defects of 4.0-, 7.0-, 50.0- and 88.0-fold, respectively, compared with the parental strain after 14 days of nutrient deprivation ( Fig. 3c , paired (two-tailed) t -test, P <0.05). Although the mazEF TA systems were induced in the NRP state, the growth kinetics of the parental and triple-mutant strains were similar for up to 40 days in the Wayne model of hypoxia ( Supplementary Fig. 5d ). Next, we investigated the growth kinetics of both the wild-type and ΔmazF3Δ9Δ6 strains in THP-1 macrophages. Compared with the parental strain, the survival of the triple-mutant strain was impaired ~4.0-fold in macrophages at day 6 post infection ( Fig. 3d , paired (two-tailed) t -test, P <0.05). These observations raise the possibility that MazF ribonucleases may contribute to the growth of Mtb in macrophages and its adaptation to conditions such as oxidative stress and nutrient deprivation. 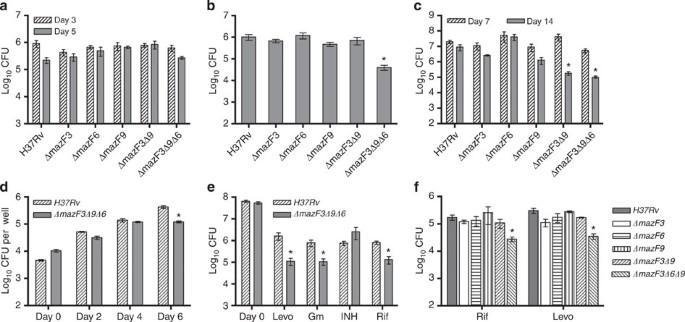Figure 3: Susceptibility of strains to various stress conditions. (a) For nitrosative stress, strains were grown until early-log phase, washed twice with MB7H9 medium at pH 5.2 and subsequently exposed to 5 mM NaNO2for either 3 or 5 days. (b) For oxidative stress, strains were exposed to 5 mM H2O2for 24 h. (c) For nutritional stress, bacilli were harvested, washed and resuspended in 1 × TBST for 7 or 14 days. At the designated time points, bacterial enumeration was performed by plating 100 μl of tenfold serial dilutions, and MB7H11 plates were incubated at 37 °C for 3–4 weeks. The data depicted are the mean±s.e. of triplicate samples and are representative of three independent experiments. Significant differences were observed for the indicated groups (paired (two-tailed)t-test, *P<0.05). (d) Effect of deletion of MazF toxins onMtbgrowth in THP-1 macrophages. THP-1 cells were infected with either the wild-type or triple-mutant strain at an multiplicity of infection of 1:1. The number of intracellular bacteria was determined by lysing macrophages in 1 × PBST and plating tenfold serial dilutions on MB7H11 plates. The data presented in this panel are the mean±s.e. of triplicate wells and are representative of two independent experiments. Significant differences were observed for the indicated groups (paired (two-tailed)t-test, *P<0.05). (e,f) Influence of the deletion of MazF toxins onMtbdrug tolerancein vitro. Wild-type and mutant strains were grown until mid-log phase and subsequently exposed to Levo, Gm, INH or Rif. At the designated time points, bacterial enumeration was performed by plating tenfold serial dilutions, and MB7H11 plates were incubated at 37 °C for 3–4 weeks. The data depicted are mean±s.e. of triplicate samples and are representative of three independent experiments. Significant differences were observed for the indicated groups (paired (two-tailed)t-test, *P<0.05). Figure 3: Susceptibility of strains to various stress conditions. ( a ) For nitrosative stress, strains were grown until early-log phase, washed twice with MB7H9 medium at pH 5.2 and subsequently exposed to 5 mM NaNO 2 for either 3 or 5 days. ( b ) For oxidative stress, strains were exposed to 5 mM H 2 O 2 for 24 h. ( c ) For nutritional stress, bacilli were harvested, washed and resuspended in 1 × TBST for 7 or 14 days. At the designated time points, bacterial enumeration was performed by plating 100 μl of tenfold serial dilutions, and MB7H11 plates were incubated at 37 °C for 3–4 weeks. The data depicted are the mean±s.e. of triplicate samples and are representative of three independent experiments. Significant differences were observed for the indicated groups (paired (two-tailed) t -test, * P <0.05). ( d ) Effect of deletion of MazF toxins on Mtb growth in THP-1 macrophages. THP-1 cells were infected with either the wild-type or triple-mutant strain at an multiplicity of infection of 1:1. The number of intracellular bacteria was determined by lysing macrophages in 1 × PBST and plating tenfold serial dilutions on MB7H11 plates. The data presented in this panel are the mean±s.e. of triplicate wells and are representative of two independent experiments. Significant differences were observed for the indicated groups (paired (two-tailed) t -test, * P <0.05). ( e , f ) Influence of the deletion of MazF toxins on Mtb drug tolerance in vitro . Wild-type and mutant strains were grown until mid-log phase and subsequently exposed to Levo, Gm, INH or Rif. At the designated time points, bacterial enumeration was performed by plating tenfold serial dilutions, and MB7H11 plates were incubated at 37 °C for 3–4 weeks. The data depicted are mean±s.e. of triplicate samples and are representative of three independent experiments. Significant differences were observed for the indicated groups (paired (two-tailed) t -test, * P <0.05). Full size image MazF ribonucleases are required for persistence in vitro Persisters constitute a phenotypic bacterial subpopulation that survives exposure to lethal drugs due to stochastic variations in the levels of global regulators and proteins involved in cellular metabolism and stress-responsive pathways. TA systems have been described as terminal effectors of bacterial persistence, because bacteria overexpressing these ribonucleases become drug tolerant by suppressing their metabolism. We investigated the contribution of MazF toxins to the persistence of Mtb on treatment with drugs with different mechanisms of action in vitro . Compared with the parental strain, a mid-log phase culture of the triple-mutant strain was 15.0-, 7.0- and 6.0-fold more susceptible to killing by exposure to Levo, Gm or Rif, respectively ( Fig. 3e , paired (two-tailed) t -test, P <0.05). The triple-mutant strain exhibited a similar persistence defect when early-log phase cultures were treated with Levo for either 7 or 14 days ( Supplementary Fig. 5e , paired (two-tailed) t -test, P <0.05). However, both the early-log and mid-log phase cultures of the wild-type and ΔmazF3Δ9Δ6 strains were similarly susceptible to INH exposure for either 7 or 14 days ( Fig. 3e and Supplementary Fig. 5e ). Interestingly, the minimum inhibitory concentration (MIC 99 ) values of the tested drugs for the various mutant strains were similar to the values obtained for the parental strain ( Supplementary Table 1 ). The MIC 99 values for Rif, Levo, ethambutol, INH and Gm were <0.05 μM, 0.78 μM, 3.125 μM, 0.78 μM and 0.2 μg ml −1 , respectively. These ribonucleases contribute synergistically to Mtb persistence, because the single and double deletions of mazF genes in the Mtb genome did not reduce the frequency of persister cell formation in vitro ( Fig. 3f ). The simultaneous deletion of 5 TA systems in E. coli has been shown to suppress fimbriae, thereby leading to inhibition of biofilm formation [7] . In contrast to the results obtained in E. coli , biofilm formation was similar in both the parental and triple-mutant strains ( Supplementary Fig. 5f ), consistent with observations in Streptococcus mutans [44] . MazF ribonucleases are essential for Mtb virulence Mtb mutant strains are categorized based on their growth characteristics in mouse, guinea pig, rabbit or non-human primate models as either severe growth in vivo (sgiv), growth in vivo (giv), persistence (per), pathology (pat) or dissemination (dis) mutants [45] . The conservation of these TA systems among members of the Mtb complex raises the possibility of their importance in virulence [24] . To better understand the role of MazF ribonucleases during host infection, we infected guinea pigs via aerosol with ~100 Mtb bacilli of either the parental strain or the ΔmazF3Δ9Δ6 strain. The parental strain exhibited logarithmic growth in the acute stage (4 weeks) followed by a slight decrease in the chronic stage (8 weeks) of infection ( Fig. 4 ). By 4 weeks post infection, ~7.0-fold reduction in the number of bacilli was observed in both the lungs and spleens of animals infected with the ΔmazF3Δ9Δ6 strain compared with animals infected with the parental strain ( Fig. 4a,b , paired (two-tailed) t -test P <0.05). However, at 8 weeks post infection, the number of colony forming units differed by 52.0- and 10.0-fold in the spleen and lungs, respectively, of guinea pigs infected with the wild-type and ΔmazF3Δ9Δ6 strains ( Fig. 4c , paired (two-tailed) t -test P <0.01; Fig. 4d , paired (two-tailed) t -test P <0.05). This reduction in bacterial counts was higher than those observed for Mtb strains lacking either mazF3 , mazF9 , Rv1246c ( relE1) , relE2 or Rv3358 ( relE3) , which maintained bacterial loads at levels comparable with those of the parental strain in murine infections [32] . 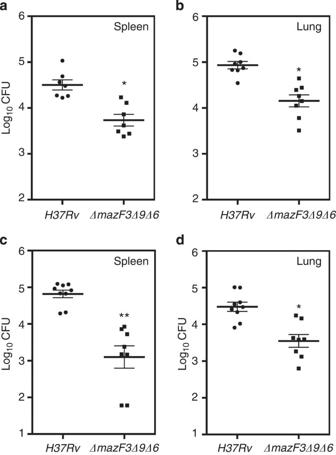Figure 4: Effect of deletion of MazF toxins on disease progression in guinea pigs. Bacillary loads in the spleens (a,c) and lungs (b,d) of guinea pigs infected with various strains were determined at 4 (a,b) and 8 weeks (c,d) post infection. At the designated time points, the spleens and lungs were homogenized in normal saline and tenfold serial dilutions were plated on MB7H11 plates, which were incubated at 37 °C for 3–4 weeks. The data shown in this panel are the mean±s.e. for each group, and each data point represents the log10CFU value for an individual animal. Significant differences were observed for the indicated groups (paired (two-tailed)t-test, **P<0.01 and *P<0.05). Figure 4: Effect of deletion of MazF toxins on disease progression in guinea pigs. Bacillary loads in the spleens ( a , c ) and lungs ( b , d ) of guinea pigs infected with various strains were determined at 4 ( a , b ) and 8 weeks ( c , d ) post infection. At the designated time points, the spleens and lungs were homogenized in normal saline and tenfold serial dilutions were plated on MB7H11 plates, which were incubated at 37 °C for 3–4 weeks. The data shown in this panel are the mean±s.e. for each group, and each data point represents the log 10 CFU value for an individual animal. Significant differences were observed for the indicated groups (paired (two-tailed) t -test, ** P <0.01 and * P <0.05). Full size image The mycobacterial growth rate in guinea pigs is not the only indicator of virulence, and studies have shown that strains with no differences in in vivo growth rates can produce infections that differ significantly by histopathological analysis [46] , [47] . Despite the reduced bacterial loads, histopathological assessments revealed that lung sections from guinea pigs infected with ΔmazF3Δ9Δ6 exhibited higher degrees of granulomatous inflammation than guinea pigs infected with the parental strain ( Fig. 5a ). At 4 weeks post infection, the lung parenchyma in these sections displayed scattered inflammatory infiltration, with the remaining areas exhibiting compensatory parenchyma ( Fig. 5b ). A more detailed quantitative analysis revealed that the total granuloma scores in lung sections from guinea pigs infected by the wild-type and ΔmazF3Δ9Δ6 strains were 15.0 and 34.0, respectively ( Fig. 5c ). However, the liver granulomas in both groups exhibited similar extents of pathological damage, with a central necrotic area surrounded by peripheral epitheloid cells ( Supplementary Fig. 6a,b ). At 8 weeks post infection, guinea pig lungs infected with the ΔmazF3Δ9Δ6 strain exhibited minimal cellular infiltration, whereas large granulomatous tissues were observed in the corresponding wild-type-infected sections ( Fig. 5d ). As shown in Fig. 5e , lung granulomas in ΔmazF3Δ9Δ6 -infected guinea pigs were non-necrotic and were composed primarily of lymphocytes, with small clusters of macrophages and epitheloid cells. A similar decrease in tissue damage was observed in the liver sections of guinea pigs infected with the ΔmazF3Δ9Δ6 strain compared with the parental strain-infected guinea pigs at 8 weeks post infection ( Supplementary Fig. 6c ). A more detailed quantitative analysis revealed that the total granuloma scores in the lung and liver sections of wild-type infected guinea pigs were 2.0-fold and 9.0-fold higher, respectively, in comparison with scores obtained in ΔmazF3Δ9Δ6 -infected guinea pigs ( Fig. 5f , paired (two-tailed) t -test P <0.05 and Supplementary Fig. 6d , paired (two-tailed) t -test P <0.01). 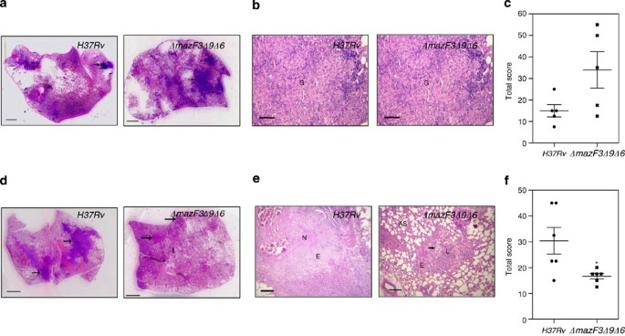Figure 5: Gross pathological and histopathological analysis of lung sections of guinea pigs infected with various strains. (a) High-resolution scanning (2,400 dpi) of lung sections from infected guinea pigs was performed at 4 weeks post infection. A representative high-resolution photomicrograph for each group is shown; granulomas in these sections are marked by arrows. Scale bar, 1.5 mm. (b) Representative photomicrographs of haematoxylin and eosin (H&E)-stained 5-μm lung sections (× 100) from infected guinea pigs at 4 weeks post infection are shown. The granulomas (G) in the lung sections from both groups predominately consisted of epitheloid cells, with very few lymphocytes. Scale bar, 100 μm. (c) Total granuloma score in H&E-stained lung sections of animals infected with the wild-type andΔmazF3Δ9Δ6strains at 4 weeks post infection. The data depicted are the mean±s.e. for each group and each data point represents the granuloma score for an individual animal. (d) High-resolution scanning (2,400 dpi) of lung sections from infected guinea pigs was performed at 8 weeks post infection. The representative lung sections from guinea pigs infected with the wild-type and triple-mutant strains depict the presence of two large coalesced and two small granulomas, respectively. Scale bar, 1.5 mm. (e) Representative photomicrographs of H&E-stained (× 40) lung sections at 8 weeks post infection. The lung sections from guinea pigs infected withΔmazF3Δ9Δ6displayed less pathological damage compared with sections from guinea pigs infected with the wild-type strain. In this panel N, E, L and AS represent necrosis, epitheloid cells, lymphocytes and alveolar space, respectively. Scale bar, 200 μm. (f) Total granuloma score in H&E-stained lung sections of animals infected with various strains at 8 weeks post infection. The data depicted in this panel are the mean±s.e for each group and each data point represents the granuloma score for an individual animal. Significant differences were observed for the indicated groups (paired (two-tailed)t-test, *P<0.05). Figure 5: Gross pathological and histopathological analysis of lung sections of guinea pigs infected with various strains. ( a ) High-resolution scanning (2,400 dpi) of lung sections from infected guinea pigs was performed at 4 weeks post infection. A representative high-resolution photomicrograph for each group is shown; granulomas in these sections are marked by arrows. Scale bar, 1.5 mm. ( b ) Representative photomicrographs of haematoxylin and eosin (H&E)-stained 5-μm lung sections (× 100) from infected guinea pigs at 4 weeks post infection are shown. The granulomas (G) in the lung sections from both groups predominately consisted of epitheloid cells, with very few lymphocytes. Scale bar, 100 μm. ( c ) Total granuloma score in H&E-stained lung sections of animals infected with the wild-type and ΔmazF3Δ9Δ6 strains at 4 weeks post infection. The data depicted are the mean±s.e. for each group and each data point represents the granuloma score for an individual animal. ( d ) High-resolution scanning (2,400 dpi) of lung sections from infected guinea pigs was performed at 8 weeks post infection. The representative lung sections from guinea pigs infected with the wild-type and triple-mutant strains depict the presence of two large coalesced and two small granulomas, respectively. Scale bar, 1.5 mm. ( e ) Representative photomicrographs of H&E-stained (× 40) lung sections at 8 weeks post infection. The lung sections from guinea pigs infected with ΔmazF3Δ9Δ6 displayed less pathological damage compared with sections from guinea pigs infected with the wild-type strain. In this panel N, E, L and AS represent necrosis, epitheloid cells, lymphocytes and alveolar space, respectively. Scale bar, 200 μm. ( f ) Total granuloma score in H&E-stained lung sections of animals infected with various strains at 8 weeks post infection. The data depicted in this panel are the mean±s.e for each group and each data point represents the granuloma score for an individual animal. Significant differences were observed for the indicated groups (paired (two-tailed) t -test, * P <0.05). Full size image TA systems are differentially induced under adverse environmental conditions such as amino acid starvation, oxidative stress and hypoxia, and in macrophages and host tissues [24] , [32] , [40] , [41] , [42] . The present study was conducted to investigate the role of MazEF TA systems in the physiology, drug-tolerance and virulence of Mtb . We observed that the overexpression of MazF3, MazF6 or MazF9 in Mtb induced a state of reversible bacteriostasis, consistent with the results of previous studies ( Fig. 1a,b ) [24] , [26] , [48] . The mycobacterial strains overexpressing these MazF toxins were viable with intact membranes under aerobic conditions. Our results are consistent with those of previous studies demonstrating that the overexpression of MazF toxins induces bacteriostasis in Staphylococcus aureus and E. coli [49] , [50] . However, in contrast to previously published studies in E. coli and Msm , the overexpression of MazF2, MazF5 or MazF7 did not affect the viability of M. bovis BCG [24] , [26] , [48] . Such variations could be due to the use of (i) different inducer-based expression systems, (ii) different host strains or (iii) vectors with different translation signals. The similarity of the growth patterns of the parental and M. bovis BCG strains overexpressing MazF1, MazF2, MazF4, MazF5, MazF7 or MazF8 was not due to a defect in the induction of these toxins. We did not observe any cross-talk between these non-cognate MazEF protein pairs, in contrast to previous reports ( Fig. 1f ) [43] . RT–PCR analysis demonstrated the differential induction of the mazEF TA systems, and under most of the conditions tested, the levels of antitoxins transcripts were lower than the levels of their cognate toxin transcripts ( Fig. 1c–e ). These differences in the transcript levels may be attributed to the differential stability of the transcripts or the expression of mazF is driven from multiple promoters. Similar post-transcriptional regulation of TA modules has also been observed in E. coli and during infection of macrophages and mice with Mtb [32] , [41] , [42] . To further elucidate the role of MazF3, MazF6 and MazF9 in Mtb physiology, we constructed various mutant strains devoid of activity associated with these ribonucleases. The replacement of the MazF3, MazF6 and MazF9 open-reading frames with antibiotic resistance genes in the respective mutant strain(s) was confirmed by both PCR and RT–PCR analysis ( Fig. 2 ). We also observed posttranscriptional regulation of mazEF6 and mazEF9 TA systems via degradation of mazE6 and mazE9 mRNA by their cognate toxins. In addition, there is a possibility that MazF toxin in complex with their cognate antitoxin can regulate transcription from their own promoter as reported in the case of MazEF6 (ref. 51 ). To establish a successful infection, Mtb must adapt to acidic, nitrosative, oxidative, nutrient-limiting and low-oxygen conditions encountered in the host. We have demonstrated that these MazF toxins are dispensable for Mtb growth in vitro , as well as for its adaptation to nitrosative stress ( Fig. 3a ) or low-oxygen conditions. The MazEF TA systems may act synergistically with other TA systems to adapt to these conditions. However, these MazF toxins contribute cumulatively to the ability of Mtb to adapt to oxidative stress conditions ( Fig. 3b ). The enhanced susceptibility of the triple-mutant strain could arise from the accumulation of (i) branched chain amino acids, as reported for a TA-deficient strain of Msm [38] , or (ii) transcription factors known to repress genes involved in the adaptation to oxidative stress. Similarly, the MqsAR and PstT1 TA modules play important roles in the adaptation of E. coli to oxidative stress [52] , [53] . Consistent with our RT–PCR results, the single-, double- and triple-mutant strains exhibited significant survival defects compared with the parental strain under nutrient-limiting conditions ( Fig. 3c ). In addition, the growth of the triple-mutant strain in THP-1 macrophages was impaired, suggesting that these enzymes are required for Mtb virulence ( Fig. 3d ). Factors such as quorum sensing, cell density, nutrient starvation, diauxic carbon source transitions, environmental signals (such as heat shock, oxidative stress and DNA damage) and stringent response pathways contribute to microbial persistence in vitro [54] , [55] , [56] , [57] , [58] , [59] . TA modules that are upregulated in persisters are terminal effectors of microbial persistence [60] , [61] . Ectopic overexpression of ribonucleases (RelE and MazF toxin), HipA (a glutamyl transfer RNA synthetase protein kinase) and TisB (membrane damage protein) enhances drug tolerance in bacteria [39] , [62] , [63] , [64] . In E. coli , TA systems function synergistically, and the successive deletion of 10 TA systems progressively reduces persister cell formation in vitro [8] . In this study, we observed that MazEF TA systems are differentially induced in Mtb persisters, and simultaneous deletion of MazF3, MazF6 and MazF9 significantly reduced persister cell formation in vitro . Compared with the parental strain, the triple-mutant strain was more susceptible to killing by Levo, Gm or Rif ( Fig. 3e ). However, both the wild-type and triple-mutant strains exhibited similar susceptibilities to INH, suggesting that INH persisters are formed through a mechanism independent of MazF toxins ( Fig. 3e ). This reduction in persister cell formation was not observed in single or double deletions of MazF ribonucleases ( Fig. 3f ). In contrast to their roles in biofilm formation in E. coli , we determined that MazF ribonucleases are dispensable for Mtb biofilm formation. The pathways that are important for the adaptation of Mtb to oxidative stress and nutrient-limiting conditions are also important for virulence. The guinea pig experimental model of tuberculosis has been used extensively to evaluate TB regimens and new vaccine candidates, as well as the characterization of mycobacterial virulence factors [65] . The pulmonary granulomas that develop in guinea pigs following aerosol exposure mimic human tubercles in every respect, except cavitation. However, unlike humans, guinea pigs are inherently susceptible to infection, indicating that the immune response, which functions well to contain human infections, is deficient in guinea pigs [65] . In our guinea pig experiments, the growth of the triple-mutant strain was attenuated at both 4 and 8 weeks post infection ( Fig. 4 ). This defect was more pronounced at the later stages of infection, thereby suggesting that MazF ribonucleases enable Mtb to adapt to environmental changes associated with the onset of host adaptive immunity ( Fig. 4c,d ). The contribution of MazF toxins to Mtb pathogenesis is further supported by the significantly reduced pathology observed in lung and liver sections from guinea pigs infected with the triple-mutant strain compared with sections from guinea pigs infected by the wild-type strain ( Fig. 5 ). The growth defect was more prominent in the spleen and the liver than the lungs, indicating that MazF toxins may play a major role in the dissemination of the disease from the lungs to the spleen and liver. TA systems have also been reported to contribute to the virulence of other pathogens such as Haemophilus influenzae , Salmonella and enteropathogenic E. coli [53] , [66] , [67] . These results suggest that MazF ribonucleases enable Mtb to survive the environmental stresses (for example, oxidative and nutritional stresses) and/or immune responses encountered in the host. Based on these findings, we propose the following model for the regulation of bacterial metabolism by TA systems ( Fig. 6 ). Exposure of Mtb to various stress conditions leads to proteolytic cleavage of a subset of antitoxins. The cognate toxins are then free to degrade the existing transcripts based on their recognition sequences, leading to a reduction in bacterial metabolism. Mtb responds to this metabolic shutdown by upregulating genes known to be induced under conditions such as drug exposure, low oxygen or nutrient limitation. We speculate that the induction of the stress regulon in response to the presence of free toxins enables Mtb to remain dormant and persist in the host. The results presented in this study demonstrate that MazF toxins contribute to the ability of Mtb to (i) adapt to oxidative and nutrient-limiting conditions, (ii) become drug-tolerant and (iii) persist in the host. Future experiments include identifying cellular targets for these ribonucleases and elucidating the roles of other TA systems in Mtb physiology and virulence. In the present study, we conclude that MazF toxins act synergistically and may be appropriate targets for combating drug-tolerant and dormant bacteria. 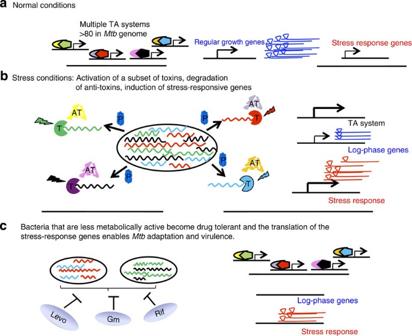Figure 6: Model proposed for the regulation of bacterial metabolism by TA systems inMtb. (a) Under normal physiological conditions, the TA complex binds and represses the transcription of its self-promoter. (b) Under stress conditions, antitoxins (AT) are cleaved by cellular proteases (P), and the presence of free toxins (T) leads to the induction of genes belonging to the stress regulon. (c) These bacteria, which have reduced metabolism and altered gene expression profiles, become drug-tolerant and are able to persist in the host. Figure 6: Model proposed for the regulation of bacterial metabolism by TA systems in Mtb . ( a ) Under normal physiological conditions, the TA complex binds and represses the transcription of its self-promoter. ( b ) Under stress conditions, antitoxins (AT) are cleaved by cellular proteases (P), and the presence of free toxins (T) leads to the induction of genes belonging to the stress regulon. ( c ) These bacteria, which have reduced metabolism and altered gene expression profiles, become drug-tolerant and are able to persist in the host. Full size image Bacterial strains and plasmids The bacterial strains and plasmids used in this study are listed in Table 1 . The E. coli strains XL-1 Blue (Stratagene, La Jolla, CA, USA) and HB-101 (Life Technologies, Carlsbad, CA, USA) were used for cloning, whereas BL-21 (λDE3, pLysS, New England Biolabs, Ipswich, MA, USA) and TB-1 cells (New England Biolabs) were used for protein expression studies. E. coli strains were cultured in Luria–Bertani broth or Luria–Bertani agar at 37 °C, 200 r.p.m. Mycobacterial strains were cultured in MB7H9 supplemented with ADS (0.81 mg ml −1 NaCl, 5 mg ml −1 BSA fraction V, 2 mg ml −1 glucose), 0.2% glycerol and 0.05% Tween-80 or minimal medium, or MB7H11 agar plates supplemented with OADS (ADS with 0.0006% v/v oleic acid) enrichment, as per standard protocols [68] . In this study, Mtb H 37 Rv and M. bovis BCG Danish were used as parental strains for the construction of various overexpression and mutant strains. Most of the antibiotics and chemicals used in the present study, unless specifically mentioned, were purchased from Sigma Aldrich (St Louis, MO, USA). Molecular biology reagents such as restriction enzymes, T4 DNA ligases and DNA polymerases were purchased from New England Biolabs or Life Technologies. The antibiotics were used at the following concentrations: kanamycin at 50 and 25 μg ml −1 for E. coli and mycobacteria, respectively; hygromycin at 150 and 50 μg ml −1 for E. coli and mycobacteria, respectively; chloramphenicol at 34 μg ml −1 for both E. coli and mycobacteria; and ampicillin at 100 μg ml −1 for E. coli . The following drugs were used in this study: Rif at 0.4 μg ml −1 , Gm at 10 μg ml −1 , Levo at 10 μg ml −1 and INH at 10 μg ml −1 . Table 1 List of strains, plasmids and phages used in the study. Full size table Protein–protein interaction and ribonuclease assays The sequences of the primers used in this study are listed in Supplementary Table 2 . For in vitro protein–protein interaction studies, genes encoding MazE antitoxins and MazF toxins were PCR amplified, sequenced and cloned into pGEX4T-1 (GE Healthcare, CT, Fairfield, USA) or pMAL-c2x (New England Biolabs), respectively. The expression of recombinant proteins in transformants was induced by addition of isopropyl β- D -galactopyranoside at a final concentration of 1 mM, followed by overnight incubation at 18 °C. Protein purification of GST-tagged antitoxins and MBP-tagged toxins from clarified bacterial lysates was performed by affinity chromatography using either glutathione Sepharose-4B (GE Healthcare) or amylose resin (New England Biolabs), according to the manufacturer’s recommendations. The purified fractions were pooled together, concentrated, dialysed overnight and stored at −80 °C. To investigate protein–protein interactions between MazF toxins and MazE antitoxins, amylose resin pre-equilibrated with binding buffer (20 mM Tris pH 8.0, 200 mM NaCl, 1 mM EDTA and 0.5% Nonidet-P40), were pre-incubated with 5 μg each of MBP-tagged and GST-tagged proteins at 4 °C with end-to-end mixing. After incubation for 2 h, the beads were subsequently washed five times with ice-cold binding buffer, and the bound protein complexes were eluted using elution buffer (20 mM Tris pH 8.0, 200 mM NaCl, 1 mM EDTA, 10 mM maltose). The protein complexes were visualized by immunoblot analysis using anti-GST antibody (1:1,000), according to the manufacturer’s recommendations. For in vitro RNA cleavage assays, linearized recombinant pGEM-T easy clones were used as templates for mRNA preparation using in vitro RNA transcription kit (Life Technologies). The synthesized mRNA was incubated with GST-tagged proteins in reaction buffer (20 mM Tris pH 7.5, 100 mM NaCl and 1 mM dithiothreitol) at 37 °C for 1 h. The reaction products were resolved on 2% agarose gels. RT–PCR studies The relative transcript levels of mazE3 , mazF3 , mazE6 , mazF6 , mazE9 and mazF9 were quantified at different growth stages or on exposure to various stress conditions or drugs as previously described [68] . For RT–PCR analysis, total mRNA was isolated using RNAeasy columns (Qiagen), treated with DNase I and complementary DNA was synthesized using Superscript III reverse transcriptase, according to standard protocols (Life Technologies). The synthesized cDNA was subjected to PCR analysis using gene-specific primers as previously described [68] . Construction of various mutant and overexpression strains Various Mtb mutant strains were constructed using the temperature-sensitive mycobacteriophage phAE87, as described previously [69] . Briefly, to generate the mutant strains, 800 bp of upstream and downstream regions flanking the gene of interest were amplified by PCR and cloned into pYUB854 flanking the desired antibiotic-resistance gene. The recombinant cosmid was subsequently packaged into phAE87 using Gigapack III packaging extract (Stratagene). Deletion of the ribonucleases from the genomes of the mutant strains was confirmed by PCR and RT–PCR analysis using gene-specific primers. The details of the plasmids used to overexpress MazF1, MazF2, MazF3, MazF4, MazF5, MazF6 and MazF9 have been described previously [32] . To construct the MazF7 and MazF8 overexpression strains, the corresponding genes were amplified by PCR and cloned into the Atc-inducible vector pTE-mcs1 . The recombinant constructs were used to transform either Mtb or M. bovis BCG by electroporation, and transformants were selected on MB7H11 plates supplemented with hygromycin. The expression of the MazF toxins in these overexpression strains was induced by adding 50 ng ml −1 Atc. The induction levels for MazF toxins in various overexpression strains were verified by RT–PCR using gene-specific primers. Bacterial viability and membrane potential studies The effect of MazF overexpression on M. bovis BCG viability was evaluated using a BacLight live/dead cell viability kit, according to the manufacturer’s recommendations (Life Technologies). Briefly, bacilli were stained with a SYTO-9/propidium iodide mix, and SYTO-9-stained live and propidium iodide-stained dead bacilli were viewed using an FV1000 Olympus confocal microscope and Fluoview software (Olympus, Tokyo, Japan). The membrane potential of various M. bovis BCG strains was calculated using a BacLight membrane potential kit, according to the manufacturer’s recommendations (Life Technologies,). The membrane potential of various mycobacterial strains was determined by measuring the ratios of red fluorescence (Ex n 485 nm/Em n 590 nm) to green fluorescence (Ex n 485 nm/Em n 528 nm) using a Biotek Synergy HT microplate reader and Gene 5 software (Biotek Instruments, Inc., Winooski, VT, USA). Mtb stress and persistence assays The growth kinetics of various strains in either MB7H9 medium or minimal medium was determined by OD 600nm measurement. The susceptibility of the parental and mutant strains to oxidative and nitrosative stress was determined as described previously [68] . To understand the role of MazF toxins in the adaptation of Mtb to nutritional stress, various strains were grown until early-log phase, washed twice with 1 × TBST and resuspended in TBST for either 7 or 14 days. For the hypoxia experiments, persistent bacilli in the non-replicating state were generated in sealed tubes and bacillary counts were determined at days 14, 28 and 40. For the in vitro drug tolerance assays, various strains were grown in MB7H9 medium until either early-log or mid-log phase and exposed to different drugs for either 7 or 14 days. For bacterial enumeration, tenfold serial dilutions were plated and MB7H11 plates were incubated at 37 °C for 3–4 weeks. The MIC 99 values of various drugs for the wild-type and mutant strains were determined using the inverted plate reader method. For biofilm formation, various strains were cultured in Sautons medium without shaking in polystyrene-coated six-well plates at 37 °C for 3–4 weeks. Macrophage infection studies The THP-1 monocyte cell line was procured from the National Centre for Cell Science, Pune, India. THP-1 cells were differentiated into adherent macrophages by adding 30 nM phorbol-12-myristate-13-acetate and seeded at a density of 5 × 10 5 per well in a 24-well plate. Macrophages were infected with various strains at a multiplicity of infection of 1:1 for 4 h, and extracellular bacilli were removed by overlaying macrophages with complete RPMI medium containing 200 μg ml −1 amikacin for 2 h. At designated time points (days 0, 2, 4 and 6 post infection), infected macrophages were lysed in 1 × PBS containing 0.1% Triton X-100, and intracellular bacteria were enumerated by plating tenfold serial dilutions on MB7H11 plates. In vivo guinea pig experiments The animal experiments were approved by the animal ethics committee of the International Centre for Genetic Engineering and Biotechnology, New Delhi, India (Approval No: ICGEB/AH/2012/1/TACF-THSTI-2). These experiments were performed in accordance with the guidelines provided by the Committee for the Purpose of Control and Supervision of Experiments on Animals (CPCSEA, Govt of India). For animal experiments, 3- to 4-week-old female guinea pigs (Hartley strain, 200–300 g) were purchased from Lala Lajpat Rai University, Hissar. To determine the contribution of MazF toxins to Mtb pathogenesis, guinea pigs were infected via the aerosol route with log-phase growing Mtb cultures (OD 600nm ~0.7–0.8). For CFU analysis, at days 1, 28 and 56 post infection, tissues were homogenized in normal saline, and tenfold serial dilutions were plated on MB7H11 plates. For histopathological analysis, liver and lung sections were fixed in 10% formalin and stained with hematoxylin and eosin. The extent of tissue damage in these sections was determined by calculating the total granuloma score and cellular infiltration as described previously [68] . Statistical analysis Prism 5 software (Version 5.01; GraphPad Software Inc., CA, USA) was used for statistical analyses and the generation of graphs. For normally distributed data, comparisons between groups were performed by a paired (two-tailed) t -test. Differences between strains were considered significant at P <0.05. How to cite this article : Tiwari, P. et al . MazF ribonucleases promote Mycobacterium tuberculosis drug tolerance and virulence in guinea pigs. Nat. Commun. 6:6089 doi: 10.1038/ncomms7059 (2015).